Tuning Piezo ion channels to detect molecular-scale movements relevant for fine touch In sensory neurons, mechanotransduction is sensitive, fast and requires mechanosensitive ion channels. Here we develop a new method to directly monitor mechanotransduction at defined regions of the cell-substrate interface. We show that molecular-scale (~13 nm) displacements are sufficient to gate mechanosensitive currents in mouse touch receptors. Using neurons from knockout mice, we show that displacement thresholds increase by one order of magnitude in the absence of stomatin-like protein 3 (STOML3). Piezo1 is the founding member of a class of mammalian stretch-activated ion channels, and we show that STOML3, but not other stomatin-domain proteins, brings the activation threshold for Piezo1 and Piezo2 currents down to ~10 nm. Structure–function experiments localize the Piezo modulatory activity of STOML3 to the stomatin domain, and higher-order scaffolds are a prerequisite for function. STOML3 is the first potent modulator of Piezo channels that tunes the sensitivity of mechanically gated channels to detect molecular-scale stimuli relevant for fine touch. Skin sensations are richly varied; contrast the flutter sensation set off by a tuning fork to the pain of a blunt impact. Many people have the ability to perceive vibrations with peak-to-peak amplitudes of just a few hundred nanometres [1] , [2] . In contrast, blunt pressure stimuli are signalled by distinct mechanosensitive afferents and are perceived as painful. Both fine and coarse mechanical stimuli are detected by a heterogeneous group of primary afferents with their cell bodies in the trigeminal and dorsal root ganglia (DRG). Virtually all sensory neurons are capable of converting mechanical stimuli into an electrical signal, a process termed mechanotransduction [3] , [4] , [5] . However, the sensitivity of the primary transduction mechanism must be scaled between different sensory neuron types to cover the range of relevant mechanosensory stimuli. The issue of dynamic range and its molecular basis has received scant attention to date. The primary transduction mechanism used to convert mechanical energy into an electrical signal in sensory neurons requires mechanosensitive ion channels, and mechanosensitive currents can be evoked in acutely isolated sensory neurons by indenting the cell soma or neurites [6] , [7] , [8] , [9] , [10] , [11] , [12] , [13] . Auditory mechanotransduction in hair cells of the inner ear also relies on mechanosensitive ion channels, and here the mechanotransduction apparatus has nanometre sensitivity for low and high frequencies. The identity of the mechanically gated ion channel for hearing is unknown. Nevertheless, the biophysical properties of hair cell mechanotransducers have been well characterized and are remarkably uniform in different hair cell types [14] . In contrast, the biophysical properties of mechanotransducers in sensory neurons are heterogeneous and may indicate the presence of more than one type of mechanosensitive ion channel [3] , [10] . Sensory neurons can be broadly classed into one of two major groups, mechanoreceptors (required for touch) and nociceptors (required for mechanical pain). It might be expected that mechanosensitive currents in nociceptors have higher displacement thresholds for activation than those found in mechanoreceptors, and there is evidence to support this idea [8] , [10] . However, existing techniques are ill-suited to address open questions about the precise mode by which mechanosensitive ion channels are gated in sensory neurons. For example, mechanosensitive channels may open on local membrane stretch or may be gated by changes in tension transferred to the channel via the cytoskeleton or via attachments to the extracellular matrix (ECM). The most common technique used to activate mechanosensitive currents in sensory neurons is indentation of the cell soma or neurite. An alternate method to activate mechanosensitive channels is to use positive or negative pressure applied to cell-attached or -excised patches of membrane [15] , [16] , [17] , [18] , [19] . However, the latter method runs the danger of removing the channel from the cytoskeletal or ECM environment in which it normally resides and is activated. There is now considerable evidence in sensory neurons that functional mechanotransduction complexes form at the cell-substrate interface and include not only the mechanically gated ion channels but also intracellular and extracellular components linked to the ECM [6] , [10] , [11] , [20] . If this model is correct, cell soma or neurite indentation represents an indirect stimulation method of the relevant transduction complexes, as force must be propagated through the entire cell to gate channels at the cell-substrate interface. The physical dimensions of the DRG neurons and neurites vary significantly [21] and there will be a viscoelastic deformation of the cell or neurite [22] on indentation. There are thus large uncertainties about the precise contact area of the probe and the area of the cell-substrate interface actually subjected to any mechanical displacement. In addition, any variation in the mechanical properties of the cells will modulate the stimulus. One fundamental consequence of these experimental limitations is that truly accurate measurements of the displacement needed to gate mechanosensitive channels in sensory neurons are missing. Here we introduce a new technique using precise movement of defined substrate areas to gate mechanosensitive channels. This technique has enabled us for the first time to measure the precise displacements required to open mechanosensitive ion channels and to study their modulation. Mouse stomatin-like protein 3 (STOML3) is a member of the stomatin-domain family of proteins that, like its Caenorhabditis elegans orthologue MEC-2, is required for normal mechanotransduction in touch receptors [20] , [23] , [24] . The molecular mechanisms by which this protein regulates mechanosensitive channels are, however, unknown. Recently, the Piezo proteins have been identified as true mechanosensitive ion channels implicated in sensory mechanotransduction, both in rat DRG neurons and in nociceptors of fruit fly larvae [25] , [26] , [27] . We show that a subpopulation of mechanoreceptors have native mechanosensitive currents that are ultrasensitive to tiny substrate deflections (<13 nm) for which STOML3 is required. Furthermore, in heterologous systems STOML3 can tune Piezo-mediated currents to molecular-scale deflections (~10 nm), as observed in native sensory neurons, and we identify key residues in the STOML3 molecule required for the modulation. Thus, STOML3 can tune the sensitivity of sensory neurons to mechanical stimuli and this molecular mechanism may in part account for the wide range of sensitivity exhibited by sensory neurons. Using pillar arrays as force transducers We developed a novel method to quantitatively study mechanoelectrical transduction at the cell-substrate interface. This method fulfils the following important design specifications: the stimulus is applied to spatially defined regions of the cell-substrate interface; the magnitude of stimulus movement can be measured with nanometre precision; and the method is compatible with stable patch-clamp recordings. To meet these experimental requirements, we cultured mouse DRG neurons on elastomeric pillar arrays cast from polydimethylsiloxane (PDMS) and applied stimuli via the substrate by deflecting a single pilus, using a piezo-driven nanomotor ( Fig. 1 ; Supplementary Movie 1 ), while monitoring fast cellular responses using a whole-cell patch clamp. 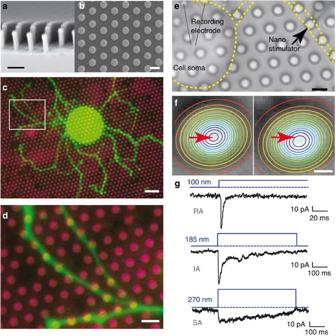Figure 1: Elastomeric pillar arrays for mechanical stimulation. (a,b) SEM images of pillar arrays; scale bars 5 μm. (c) Acutely prepared DRG neuron expressing Lifeact-mGFP (green) cultured on EHS laminin/Cy3-coated pillar arrays (magenta); scale bar 20 μm. (d) Cultured DRG neuron neurites grow across the tops of pili (similar observations made in five cells, from three transfections); scale bar 5 μm. (e) Mechanical stimuli are applied to the neuron–laminin interface by applying a series of deflections to an individual pilus while recording from the cell with a whole-cell patch clamp. Black arrow indicates pilus being moved; attached neurite is outlined in yellow; scale bar 5 μm. (f) The centre point (red arrow) is determined using a 2D-Gaussian fit of intensity values; scale bar 1 μm. (g) Nanoscale stimuli applied at the neuron–substrate interface activate RA, IA or SA currents (observations made in 23 cells). Figure 1: Elastomeric pillar arrays for mechanical stimulation. ( a , b ) SEM images of pillar arrays; scale bars 5 μm. ( c ) Acutely prepared DRG neuron expressing Lifeact-mGFP (green) cultured on EHS laminin/Cy3-coated pillar arrays (magenta); scale bar 20 μm. ( d ) Cultured DRG neuron neurites grow across the tops of pili (similar observations made in five cells, from three transfections); scale bar 5 μm. ( e ) Mechanical stimuli are applied to the neuron–laminin interface by applying a series of deflections to an individual pilus while recording from the cell with a whole-cell patch clamp. Black arrow indicates pilus being moved; attached neurite is outlined in yellow; scale bar 5 μm. ( f ) The centre point (red arrow) is determined using a 2D-Gaussian fit of intensity values; scale bar 1 μm. ( g ) Nanoscale stimuli applied at the neuron–substrate interface activate RA, IA or SA currents (observations made in 23 cells). Full size image Positive silicon masters were microfabricated and used to generate negative moulds from which pillar arrays were cast [28] ( Fig. 1a,b ). We created several different pillar geometries but found two on which sensory neurons extend neurites and most data presented here were generated using pili with a top surface area of 10.07 μm 2 and a spring constant ( k ) of 290 pN nm −1 ( Fig. 1b ; Supplementary Fig. 1 ); some experiments were carried out with thinner, more compliant ( k =6.7 pN nm −1 ) pillar arrays ( Supplementary Fig. 1 ). The calculated restoring force differed by an order of magnitude between the two pillar arrays but deflections needed to gate mechanosensitive currents in sensory neurons were comparable ( Supplementary Figs 1 and 3 ), suggesting that deflection and not force is the most relevant physical parameter [29] . The tops of the pili were coated with EHS laminin (hereafter called laminin), a substrate supportive of neurite outgrowth from DRG cells and permissive for mechanotransduction [6] . Within 24 h of plating, DRG neurons attach and establish neuritic trees with cell-substrate contact points restricted to the tops of the pili ( Fig. 1c,d ). We monitored neurite growth over the pili either by filling single cells with the fluorescent dye Lucifer Yellow or by transfecting cells with plasmids encoding Lifeact-eGFP to label actin [21] . To generate stimulus–response curves, a series of deflections were applied to a single pilus using a piezo-driven, heat-polished, glass tip and the resulting currents were recorded ( Fig. 1e ). For each data point, the deflection of the pilus was calculated from bright-field images taken before, during and after the stimulus: as each pilus acts as a light guide, the centre of the pilus could be calculated from a two-dimensional Gaussian fit of intensity values and the centre points from successive images were compared ( Fig. 1f ). The positions of adjacent pili were monitored to ensure that no more than one pilus moved. As in previous studies using cell indentation, three types of mechanosensitive currents could be evoked: the rapidly adapting (RA, inactivation time constant <5 ms); intermediate adapting (IA, inactivation time constant 5–50 ms); or slowly adapting (SA, little inactivation within 200 ms) currents (example current traces, Fig. 1g ). Soma and neurite indentation versus substrate deflection Very small movements of individual pili evoked robust and fast mechanosensitive currents. In contrast to soma and neurite indentation, we could generate these currents with considerably smaller stimulus magnitudes; as little as 10 nm for pillar arrays compared with 200–750 nm for neurite indentation [6] , [10] , [20] and 1–9 μm for soma indentation [7] , [8] , [12] ( Fig. 2a ). The dramatically lower deflection thresholds found for mechanotransduction on pili support the idea that substrate deflection allows the most direct activation of mechanosensitive channels. We asked whether DRG neurons responded to mechanical stimuli with a single current type or with heterogeneous currents. We found that soma indentation results in a single current type in most cells, with some cells responding to multiple stimuli with two distinct current types. In contrast, in neurons where stimuli were applied by neurite indentation or pillar deflection significantly, more cells responded to multiple stimuli with more than one current type ( Fig. 2b ). This observation suggests that multiple current types may be present, but are not observed with the commonly used soma indentation technique. In addition, the smaller displacements necessary to gate mechanosensitive currents suggest that the mechanosensitive ion channels are primarily activated at the cell-substrate interface ( Fig. 2c ). 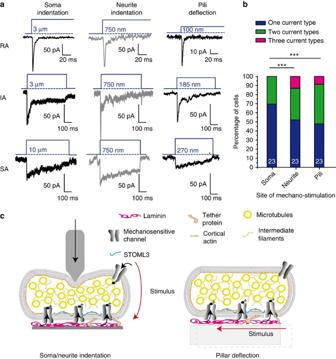Figure 2: Comparing modes of mechanical stimulation. (a) RA, IA and SA currents were observed on mechanical indentation of the soma, neurites or on deflection of a neurite-bound pilus. (b) On neurite indentation and pillar deflection, a higher variability was observed in the current types measured within a single cell (χ2test; ***P<0.001). Data collected from 23 cells in all three conditions; soma and neurite indentation represent matched data; pillar deflection is data from a separate set of cells. (c) Schematic representation of mechanical stimulation. Cell indentation studies require propagation of the physical stimulus via the cell to the cell-substrate interface. In contrast, deflecting a single pilus allows a defined stimulus to be applied directly at localized cell–matrix contacts. Figure 2: Comparing modes of mechanical stimulation. ( a ) RA, IA and SA currents were observed on mechanical indentation of the soma, neurites or on deflection of a neurite-bound pilus. (b) On neurite indentation and pillar deflection, a higher variability was observed in the current types measured within a single cell ( χ 2 test; *** P <0.001). Data collected from 23 cells in all three conditions; soma and neurite indentation represent matched data; pillar deflection is data from a separate set of cells. ( c ) Schematic representation of mechanical stimulation. Cell indentation studies require propagation of the physical stimulus via the cell to the cell-substrate interface. In contrast, deflecting a single pilus allows a defined stimulus to be applied directly at localized cell–matrix contacts. Full size image Quantification of mechanosensitivity in sensory neurons We next classified sensory neurons based on a combination of action potential (AP) characteristics and mechanotransduction thresholds. Sensory fibres innervating the skin can be broadly classified as nociceptors with high mechanical thresholds appropriate for pain sensing and mechanoreceptors with low thresholds necessary for light touch [5] . The DRG neurons that give rise to these different afferent fibres are also referred to as nociceptors and mechanoreceptors. We asked whether these two subpopulations of DRG neurons differed in terms of threshold for mechanotransduction. Mechanoreceptors have a distinctive narrow AP, and these cells possessed fast and sensitive RA or IA currents with deflection thresholds of as little as a few nanometres ( Fig. 3a,b ). The kinetics of mechanosensitive currents in mechanoreceptors was similar, but not identical to those found using cell indentation ( Supplementary Fig. 2 ; Supplementary Table 1 ). Nociceptors, classified by their broad and humped AP [12] , [30] , [31] , [32] , possessed RA, IA and SA currents that had significantly higher deflection thresholds compared with currents found in mechanoreceptors ( Fig. 3b ). The latency between the movement of a pilus and activation of the current was significantly longer in nociceptors compared with that in mechanoreceptors ( Fig. 3c ). This indicates that the differences in mechanical threshold of mechanoreceptor and nociceptor sensory fibres can be, in part, explained by differences in the threshold for mechanotransduction in individual neurons. We noticed that there was substantial variability in the stimulus–response curves of putative mechanoreceptors ( Fig. 3b ). In fact, two types of mechanoreceptors could be distinguished on the basis of their AP configuration [32] and mechanosensitive current sensitivity (see Supplementary Fig. 3 for single cell examples). Type I cells exhibited very narrow APs (<0.7 ms) with short after-hyperpolarization times (<4 ms) and type II cells displayed wider APs (>0.7 ms) with longer after-hyperpolarization times (>4 ms) ( Fig. 3d,e ). Type I cells exhibited predominantly RA currents with small amplitudes and high deflection thresholds ( Fig. 3f,g ), whereas type II cells displayed large amplitude, ultrasensitive RA and IA currents ( Fig. 3f,g ). Type II mechanoreceptors typically exhibited mechanosensitive currents to pili deflections of around 10 nm ( Fig. 3f ; Supplementary Fig. 3 ). In order to compare between cell types, we binned the data by stimulus magnitude (0–10, 10–50, 50–100, 100–250, 250–500 and 500–1,000 nm) and averaged the current amplitudes within each bin for each cell. We found that type II mechanoreceptors exhibited significantly larger currents than those observed in type I mechanoreceptors in the deflection ranges 0–10, 10–50 and 50–100 nm ( Fig. 3f ; Supplementary Table 2 ). The current amplitudes could also be modelled by a Boltzmann fit, and this analysis approximates the deflection amplitude for half-maximal activation to be 63 nm for type I and just 10 nm for type II mechanoreceptors ( Supplementary Fig. 3 ). The time constant of current activation, τ 1 , did not differ ( Fig. 3i ); however, because type II cells displayed both RA and IA currents ( Fig. 3g,h ), the mean time constant of current inactivation, τ 2 , was significantly longer (28.5±1.2 ms) (41 currents from 8 cells) compared with the mostly RA currents found in type I cells (8.2±1.2 ms) (71 currents from 8 cells) (Mann–Whitney U -test, P <0.001) ( Supplementary Table 1 ). There is thus heterogeneity in mechanoreceptor sensitivity with type II cells exhibiting extraordinarily high sensitivity. This finding suggests that the heterogeneity in the sensitivity of mechanoreceptor fibres can be explained by intrinsic differences in mechanotransducer sensitivity. In fact, type II cells possessed APs that were most similar to those of D-hair receptors measured in vivo [31] , [32] . D-hair receptors are ultrasensitive skin mechanoreceptors with mechanical thresholds at least an order of magnitude lower than those of other mechanoreceptors—for example, rapidly adapting mechanoreceptors [3] , [33] , [34] . 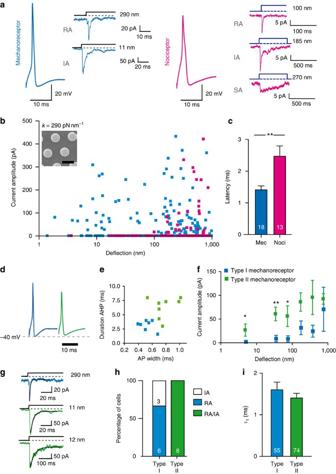Figure 3: Mechanically gated currents in mechanoreceptors and nociceptors. (a) Mechanically gated currents in mechanoreceptors (narrow AP, no hump in the falling phase) were exclusively transient RA and IA currents; in nociceptors (broad APs, hump on falling phase) RA, IA and SA currents were observed. (b) A stimulus–response plot of individual data points (blue–mechanoreceptors,n=243 data points/17 cells; magenta–nociceptors,n=110 data points/13 cells) collected on array withk=290 pN m−1(insert: SEM image of pillar array, scale bar 5 μm). (c) The latency of channel gating was significantly shorter in mechanoreceptors (n=18) versus nociceptors (n=13, Student’st-test, **P<0.01). (d,e) Mechanoreceptor APs can be classed into two additional subgroups, type I (blue) and type II (green), based on width (full-width at half-maximum) and duration of recovery after hyperpolarization. (f) Binned data indicate the higher sensitivity of type II compared with type I mechanoreceptors; current amplitudes were averaged for each bin and averages compared (type I:n=9 cells; type II:n=8 cells). To test for significance, Student'st-test was used; data are displayed as mean±s.e.m. (g) Representative currents from type I mechanoreceptors (blue trace; black line indicatesτ2fit, 2 ms) and for type II mechanoreceptors (green traces; black line indicatesτ2fit, 5.0 ms and 49). (h) Individual type I mechanoreceptors displayed either exclusively RA currents or exclusively IA currents. A mixture of both RA and IA currents was observed in individual type II mechanoreceptors. (i) Activation time constant (τ1) of mechanotransduction currents (n=55 currents, 9 type I cells; 74 currents, 8 type II cells), presented as mean±s.e.m. Data obtained for cells cultured on arrays wherek=290 pN nm−1. Figure 3: Mechanically gated currents in mechanoreceptors and nociceptors. ( a ) Mechanically gated currents in mechanoreceptors (narrow AP, no hump in the falling phase) were exclusively transient RA and IA currents; in nociceptors (broad APs, hump on falling phase) RA, IA and SA currents were observed. ( b ) A stimulus–response plot of individual data points (blue–mechanoreceptors, n =243 data points/17 cells; magenta–nociceptors, n =110 data points/13 cells) collected on array with k =290 pN m −1 (insert: SEM image of pillar array, scale bar 5 μm). ( c ) The latency of channel gating was significantly shorter in mechanoreceptors ( n =18) versus nociceptors ( n =13, Student’s t -test, ** P <0.01). ( d , e ) Mechanoreceptor APs can be classed into two additional subgroups, type I (blue) and type II (green), based on width (full-width at half-maximum) and duration of recovery after hyperpolarization. ( f ) Binned data indicate the higher sensitivity of type II compared with type I mechanoreceptors; current amplitudes were averaged for each bin and averages compared (type I: n =9 cells; type II: n =8 cells). To test for significance, Student's t -test was used; data are displayed as mean±s.e.m. ( g ) Representative currents from type I mechanoreceptors (blue trace; black line indicates τ 2 fit, 2 ms) and for type II mechanoreceptors (green traces; black line indicates τ 2 fit, 5.0 ms and 49). ( h ) Individual type I mechanoreceptors displayed either exclusively RA currents or exclusively IA currents. A mixture of both RA and IA currents was observed in individual type II mechanoreceptors. ( i ) Activation time constant ( τ 1 ) of mechanotransduction currents ( n =55 currents, 9 type I cells; 74 currents, 8 type II cells), presented as mean±s.e.m. Data obtained for cells cultured on arrays where k =290 pN nm −1 . Full size image STOML3 is required for molecular-scale sensitivity We next studied the role of STOML3, an integral membrane protein orthologous to MEC-2 from C. elegans [20] , [24] , [35] , [36] , necessary for normal touch-driven behaviour in the mouse. The behavioural deficit in stoml3 −/− mice can be attributed to mechanical insensitivity of a subset of mechanoreceptor fibres. We first transfected acutely prepared DRG neurons with a plasmid encoding STOML3-mGFP and found that the protein accumulated at the pili–neurite contact points as seen in an epifluorescence image ( Fig. 4a,b ), further supporting the hypothesis that mechanotransduction channel complexes form at the cell-substrate interface. In neurite-indentation experiments (stimulus magnitude 750 nm) with stoml3 −/− mouse DRG neurons, 36% of neurons lacked mechanosensitive currents [20] ; however, all 25 stoml3 −/− neurons studied here exhibited mechanosensitive currents on pillar deflection. This clearly demonstrates that the presence of STOML3 is not an absolute prerequisite for the formation of a functional mechanosensitive complex and suggests that the pillar array method allows us to measure high-threshold mechanosensitive currents not detectable with indentation. We classified the stoml3 −/− neurons as type I or type II mechanoreceptors or as nociceptors on the basis of AP configuration, and binned and averaged the stimulus–response data, as for wild-type cells. We found no significant difference in response to mechanical stimuli between type I mechanoreceptors from C57Bl/6 mice versus stoml3 −/− mice ( Fig. 4d ; Supplementary Fig. 4 ), a finding consistent with the preserved mechanosensitivity of many stoml3 −/− mechanoreceptor fibres [20] . In contrast, at smaller deflections (0–10, 10–50 and 50–100 nm), currents measured in type II mechanoreceptors from stoml3 −/− mice were almost absent compared with those observed in control neurons ( Fig. 4e ; Supplementary Fig. 4 ). In addition, within the deflection range of 100–250 nm, nociceptors from stoml3 −/− mice produced significantly smaller currents than those observed in nociceptors isolated from control mice ( Fig. 4f ) (See Supplementary Table 2 for a summary of statistics). When stimulus–response functions were approximated from Boltzmann fits of the data for type II mechanoreceptors and nociceptors, we noted a substantial increase of around fourfold in the deflection needed for half-maximal activation of the currents in stoml3 −/− neurons, compared with control ( Supplementary Fig. 4 ). The latencies for RA and IA currents were slightly longer in stoml3 −/− neurons than in control neurons ( Supplementary Fig. 4 ). SA currents in stoml3 −/− nociceptors had distinctly slower latencies and activation kinetics ( τ 1 ), and a 10–40-fold slowing down in both parameters ( Supplementary Fig. 4 ). These data suggest that the primary function of STOML3 may be to facilitate the transfer of force to mechanically gated channels. 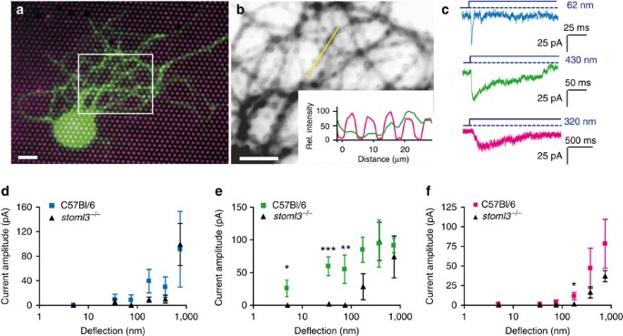Figure 4: Mechanotransduction currents in DRG neurons fromstoml3−/−mice. (a) Acutely isolated DRG neurons expressing STOML3-mGFP (green) cultured on a pillar array coated with EHS laminin/Cy3 (magenta); scale bar 20 μm. (b) STOML3-mGFP is targeted preferentially to contact points; the insert indicates line scan of intensity corresponding to the yellow line (similar observations made in eight cells, from three transfections, on eight pillar arrays); scale bar 20 μm. (c) Instoml3−/−DRG neurons, we observed RA, IA and SA currents. (d–f) All data were binned into stimulus sizes and current amplitudes were averaged for each bin and compared between C57Bl/6 mice andstoml3−/−mice. Data are displayed as mean±s.e.m. (d) Type I mechanoreceptors from C57Bl/6 mice (n=9 cells) versusstoml3−/−mice (n=7 cells). (e) Type II mechanoreceptors isolated from C57Bl/6 mice (n=8 cells) versusstoml3−/−mice (n=8 cells). (f) Nociceptors from C57Bl/6 mice (n=13 cells) versusstoml3−/−mice (n=9 cells). To test for significance Student'st-test was used; *P<0.05, **P<0.01, ***P<0.001. Data were obtained for cells cultured on arrays wherek=290 pN nm−1. Figure 4: Mechanotransduction currents in DRG neurons from stoml3 −/− mice. ( a ) Acutely isolated DRG neurons expressing STOML3-mGFP (green) cultured on a pillar array coated with EHS laminin/Cy3 (magenta); scale bar 20 μm. ( b ) STOML3-mGFP is targeted preferentially to contact points; the insert indicates line scan of intensity corresponding to the yellow line (similar observations made in eight cells, from three transfections, on eight pillar arrays); scale bar 20 μm. ( c ) In stoml3 −/− DRG neurons, we observed RA, IA and SA currents. ( d – f ) All data were binned into stimulus sizes and current amplitudes were averaged for each bin and compared between C57Bl/6 mice and stoml3 −/− mice. Data are displayed as mean±s.e.m. ( d ) Type I mechanoreceptors from C57Bl/6 mice ( n =9 cells) versus stoml3 −/− mice ( n =7 cells). ( e ) Type II mechanoreceptors isolated from C57Bl/6 mice ( n =8 cells) versus stoml3 −/− mice ( n =8 cells). ( f ) Nociceptors from C57Bl/6 mice ( n =13 cells) versus stoml3 −/− mice ( n =9 cells). To test for significance Student's t -test was used; * P <0.05, ** P <0.01, *** P <0.001. Data were obtained for cells cultured on arrays where k =290 pN nm −1 . Full size image Modulation of Piezo1-mediated currents by STOML3 There has been debate over the molecular identity of stretch-activated channels in mammalian cells [18] , but it is now clear that the Piezo proteins can form true mechanosensitive channels [25] , [26] . Therefore, we next tested the effects of STOML3 on Piezo1-mediated currents in N2a neuroblastoma cells. N2a cells were grown on uncoated pillar arrays and transfected with a plasmid encoding Lifeact-mCherry ( Fig. 5a ). In control N2a cells, pillar deflections evoked robust mechanosensitive currents with a surprising diversity of inactivation kinetics ( Fig. 5b ), including rapidly inactivating currents and essentially non-inactivating currents ( Fig. 5b ; Supplementary Table 3 ); we could find no systematic relationship between stimulus amplitude and inactivation kinetics (data not shown), but a similar behaviour for Piezo1 has been noted [19] . Compared with DRG neurons, relatively large pillar deflections were required to activate the N2a mechanosensitive current (most often >200 nm) ( Fig. 5c ; see Supplementary Fig. 5 for all individual data points). However, this stimulus size is considerably smaller than that required for channel gating using cell indentation in the same cell type (>5 μm) [26] . Using microRNA (miRNA)-mediated reduction of Piezo1 expression, we could demonstrate an almost complete loss of mechanically gated currents observed within our stimulus range (0–1,000 nm) ( Fig. 5c ), clearly demonstrating that the currents observed on pillar deflection are mediated by the same channels measured with cell indentation. 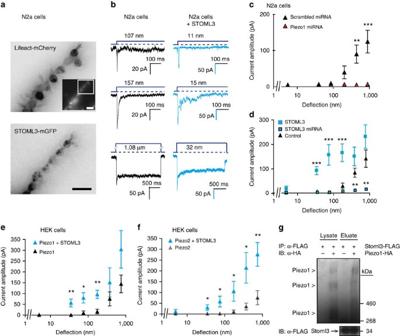Figure 5: STOML3 increases Piezo1 and Piezo2 sensitivity. (a) Inverted epifluorescence images of N2a neuroblastoma cells expressing Lifeact-mCherry and STOML3-mGFP cultured on uncoated, PDMS pillar arrays (similar observations were made in 26 cells from 7 transfections (lifeAct) and in 19 cells from 10 transfections (STOML3-mGFP)). Inset is an overview of Lifeact-mCherry signal in an individual cell; scale bars, 10 μm. (b) In individual cells, mechanically gated currents with variable kinetics were observed: black traces N2a control cells; blue traces N2a cells overexpressing STOML3-mGFP. (c–f) Stimulus–response data were binned and weighted by cell, and displayed as mean±s.e.m. and compared using Student’st-test where *P<0.05, **P<0.01, ***P<0.001. (c) When endogenous Piezo1 was knocked down with miRNA (100 measurements, 10 cells) mechanosensitivity was significantly reduced compared with control cells treated with scrambled miRNA (145 measurements, 12 cells), Two-way analysis of variance (P<0.001), with Bonferroni post-tests (**P<0.01). (d) Current amplitudes were detected with stimuli much less than 100 nm in N2a cells overexpressing STOML3-mGFP (n=19 cells) compared with control cells (n=26 cells), and knockdown of endogenous STOML3 messenger RNA led to a strong reduction in current amplitudes below control levels (**P<0.01; data compared with miRNA controls plotted in panelc). (e,f) Stimulus–response data of mechanically gated currents in HEK-293 cells expressing Piezo1 (e) or Piezo2 (f) in the presence or absence of STOML3. As seen in N2a cells, the presence of STOML3 dramatically increased Piezo channel-mediated mechanosensitivity in HEK-293 cells. (g) Co-immunoprecipitation of Piezo1 with STOML3 pulldown in HEK-293 cells. Experiment was repeated six times, and in each case bands corresponding to Piezo proteins were detected in eluates from STOML3 pulldown. Figure 5: STOML3 increases Piezo1 and Piezo2 sensitivity. ( a ) Inverted epifluorescence images of N2a neuroblastoma cells expressing Lifeact-mCherry and STOML3-mGFP cultured on uncoated, PDMS pillar arrays (similar observations were made in 26 cells from 7 transfections (lifeAct) and in 19 cells from 10 transfections (STOML3-mGFP)). Inset is an overview of Lifeact-mCherry signal in an individual cell; scale bars, 10 μm. ( b ) In individual cells, mechanically gated currents with variable kinetics were observed: black traces N2a control cells; blue traces N2a cells overexpressing STOML3-mGFP. ( c – f ) Stimulus–response data were binned and weighted by cell, and displayed as mean±s.e.m. and compared using Student’s t -test where * P <0.05, ** P <0.01, *** P <0.001. ( c ) When endogenous Piezo1 was knocked down with miRNA (100 measurements, 10 cells) mechanosensitivity was significantly reduced compared with control cells treated with scrambled miRNA (145 measurements, 12 cells), Two-way analysis of variance ( P <0.001), with Bonferroni post-tests (** P <0.01). ( d ) Current amplitudes were detected with stimuli much less than 100 nm in N2a cells overexpressing STOML3-mGFP ( n =19 cells) compared with control cells ( n =26 cells), and knockdown of endogenous STOML3 messenger RNA led to a strong reduction in current amplitudes below control levels (** P <0.01; data compared with miRNA controls plotted in panel c ). ( e , f ) Stimulus–response data of mechanically gated currents in HEK-293 cells expressing Piezo1 ( e ) or Piezo2 ( f ) in the presence or absence of STOML3. As seen in N2a cells, the presence of STOML3 dramatically increased Piezo channel-mediated mechanosensitivity in HEK-293 cells. ( g ) Co-immunoprecipitation of Piezo1 with STOML3 pulldown in HEK-293 cells. Experiment was repeated six times, and in each case bands corresponding to Piezo proteins were detected in eluates from STOML3 pulldown. Full size image Upon overexpression, the STOML3 protein was targeted to the cell–pilus contact points ( Fig. 5a ), and we observed a dramatic decrease in the deflection threshold for the Piezo1 currents, with robust currents evoked with deflections as small as 10 nm. Cells overexpressing STOML3 also exhibited significantly larger currents at smaller deflections, compared with control cells ( Fig. 5d ; Supplementary Table 4 ). Using quantitative PCR, we found low levels of endogenous STOML3 messenger RNA in N2a cells and miRNA-mediated knockdown of endogenous STOML3 dramatically reduced Piezo1 currents to pili deflections up to 1,000 nm compared with controls ( Fig. 5d ; Supplementary Fig. 5 ; Supplementary Table 4 ). We next directly tested whether STOML3 could modulate both Piezo1 and Piezo2 currents by heterologously expressing these channels with STOML3 in HEK-293 cells. Using pillar arrays, we could show that both Piezo1 and Piezo2 currents exhibited dramatically reduced deflection thresholds in the presence of STOML3 ( Fig. 5e,f ; Supplementary Fig. 5 ; Supplementary Tables 4 and 5 ). Robust channel gating was observed with molecular-scale pillar deflections similar in magnitude to those described for the most sensitive DRG neurons. Thus, STOML3 is a potent modulator of both Piezo1 and Piezo2 channels. We also carried out biochemical studies to ask whether there is a physical interaction between STOML3 and Piezo proteins. Both Piezo1 and Piezo2 proteins were found to co-precipitate with STOML3 after overexpression in HEK-293 cells ( Fig. 5g ; Supplementary Figs 5–7 ); we could detect HA-tagged Piezo1 bands in the eluate only when STOML3 was present. Interestingly, the Piezo1-positive bands detected from the immunoprecipitate appeared to represent extremely large protein complexes (>0.5 MDa) similar in size to Piezo1 proteins in SDS-polyacrylamide gel electrophoresis gels after chemical crosslinking [25] . We next determined whether the STOML3-dependent sensitization is specific to STOML3, or is a general feature of stomatin-domain proteins. We studied the effect of overexpression of stomatin, STOML1 (found in mammalian DRG neurons [36] ), podocin (found in mammalian podocytes [37] ) and MEC-2 (required for gentle body touch in C. elegans ) on mechanosensitive currents in N2a cells. No significant differences were detected in the sensitivity or the kinetics of the mechanically gated currents after overexpression of stomatin, STOML1 or MEC-2 ( Supplementary Fig. 8 ; Supplementary Tables 3 and 4 ). A mild but statistically significant effect of podocin overexpression was found only for deflections between 50 and 100 nm compared with control cells ( Supplementary Fig. 8 ; Supplementary Tables 3 and 4 ). Thus, the tuning of mechanotransduction sensitivity in N2a cells is not a general property of stomatin-domain proteins. However, we noticed that successive suprathreshold stimuli led to a steady desensitization of mechanosensitive currents in N2a cells ( Fig. 6a,b ), in a localized manner (that is, at a single pilus). Stimulation of a new pilus contacted by the same cell initially produced mechanosensitive currents of normal magnitude. In contrast, this desensitization phenomenon was considerably attenuated in N2a cells overexpressing STOML3 or STOML1, but not in cells overexpressing MEC-2, podocin or stomatin ( Fig. 6b–f ). Thus, the stomatin-domain proteins STOML1 and STOML3 have a potent effect in preventing short-term desensitization of Piezo currents dependent on prior mechanical stimulation. 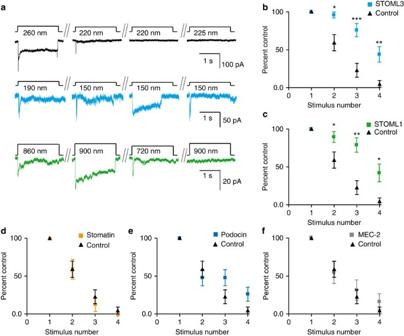Figure 6: Desensitization of mechanosensitive currents in N2a cells is prevented by STOML3 and STOML1. (a) Example traces from successive pillar deflections in control N2a cells (black traces), in N2a cells overexpressing STOML3-mGFP (cyan traces) or STOML1-mCherry (green traces). Stimuli were applied ~5 s apart. (b–e) Successive suprathreshold stimuli led to current desensitization in N2a cells (n=22 stimulation points). However, when either (b) STOML3 (n=25 stimulation points) or (c) STOML1 (n=19 stimulation points) is present, mechanosensitive currents do not desensitize as fast as controls; two-way analysis of variance (P<0.001). In addition, Bonferroni post-tests indicate that the probability of measuring a current in response to the second, third and fourth suprathreshold stimuli is significantly higher in those cells overexpressing STOML3 or overexpressing STOML1 (*P<0.05, **P<0.01, ***P<0.001). This desensitization is not modulated in the presence of (d) stomatin (n=15 stimulation points), (e) podocin (n=23 stimulation points) or (f) MEC-2 (n=13 stimulation points). Data were obtained for cells cultured on arrays wherek=290 pN nm−1. Control data are re-plotted in each panel for comparison, all data presented as mean±s.e.m. Figure 6: Desensitization of mechanosensitive currents in N2a cells is prevented by STOML3 and STOML1. ( a ) Example traces from successive pillar deflections in control N2a cells (black traces), in N2a cells overexpressing STOML3-mGFP (cyan traces) or STOML1-mCherry (green traces). Stimuli were applied ~5 s apart. ( b – e ) Successive suprathreshold stimuli led to current desensitization in N2a cells ( n =22 stimulation points). However, when either ( b ) STOML3 ( n =25 stimulation points) or ( c ) STOML1 ( n =19 stimulation points) is present, mechanosensitive currents do not desensitize as fast as controls; two-way analysis of variance ( P <0.001). In addition, Bonferroni post-tests indicate that the probability of measuring a current in response to the second, third and fourth suprathreshold stimuli is significantly higher in those cells overexpressing STOML3 or overexpressing STOML1 (* P <0.05, ** P <0.01, *** P <0.001). This desensitization is not modulated in the presence of ( d ) stomatin ( n =15 stimulation points), ( e ) podocin ( n =23 stimulation points) or ( f ) MEC-2 ( n =13 stimulation points). Data were obtained for cells cultured on arrays where k =290 pN nm −1 . Control data are re-plotted in each panel for comparison, all data presented as mean±s.e.m. Full size image STOML3 structure–function analysis We next asked whether oligomerization of STOML3 is important for its function in tuning mechanosensitivity. Stomatin, the closest relative of STOML3, forms dimers, and mutations that disrupt dimerization interfere with stomatin-mediated modulation of acid-sensing ion channels [38] . As such, we introduced a mutation into STOML3 at the orthologous position predicted to disrupt dimerization (V190P). We confirmed that STOML3-V190P exhibited reduced oligomerization in comparison with STOML3 using bimolecular fluorescence complementation assays (BiFC) [39] , [40] ( Fig. 7 ; Supplementary Fig. 9 ). The STOML3-V190P protein did not sensitize mechanically gated currents in N2a cells, and the measured currents did not differ significantly from those in wt N2a cells ( Fig. 7a ; Supplementary Table 4 ). STOML3 function is thus, in part, dependent on its ability to properly oligomerize. Despite the fact that MEC-2 did not modulate Piezo1 currents in N2a cells, we tested whether residues important for MEC-2 function are also important in STOML3 function. The u64 mec-2 allele has severe effects on gentle body touch in C. elegans , as a result of a missense mutation (R184C) at a residue conserved in mammalian stomatin-domain proteins. The corresponding Arg in STOML3, R90, is predicted to be present at an interaction surface in the stomatin domain named interface-2 (refs 38 , 41 ). Using BiFC, we analysed oligomerization of two sets of mutations designed to disrupt interface-2: STOML3-R90A and STOML3-LR89,90EE. We found that both mutations decreased the BiFC signal, and both mutations essentially abolished STOML3 modulation of mechanosensitive currents in N2a cells ( Fig. 7a,c ; Supplementary Fig. 9 ; Supplementary Table 4 ). Mutations at interface-2 also severely altered the intracellular distribution of the protein as we observed virtually no vesicular localization as seen with wild-type protein and described by us in sensory neurons [40] ( Fig.7b ). This phenotype has a striking parallel in C. elegans where the orthologous mutation leads to a mis-localization of MEC-2 (ref. 41 ). However, a fraction of the fluorescently labeled STOML3-R90A and STOML3-LR89,90EE proteins did appear to reach the membrane ( Fig.7b ). We have previously shown that stomatin, carrying a mutation at the same position, does retain some modulatory activity on ASIC3-mediated currents [38] , indicating that it can reach the plasma membrane. Some stomatin-domain proteins, including MEC-2, bind cholesterol [37] , [42] and one of the MEC-2 alleles found to abolish cholesterol binding (P134S) has a strong effect on touch-driven behaviour in the worm. The P134S MEC-2 variant shows impaired activity in modulating MEC-4/MEC-10 ion channels [37] , [42] . Mutation of the orthologous proline in STOML3 (P40S) leads to STOML3 mis-localization predominantly to the cytoplasmic compartment; yet this mutant is still fully active in modulating ASIC2a channels, suggesting that a fraction of this variant must still reach the plasma membrane [40] . In contrast, the STOML3-P40S protein lost its ability to modulate the threshold of Piezo1 currents in N2a cells ( Fig. 7a ). Thus, STOML3 modulation of ASIC currents is separable from its powerful modulatory effects on mechanosensitive currents. 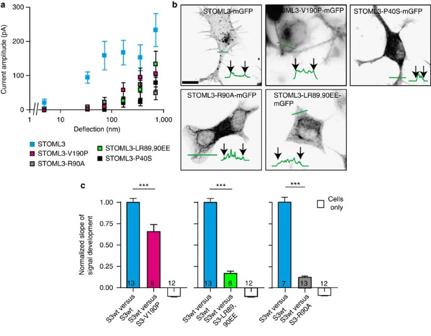Figure 7: Residues required for oligomerization and correct localization are necessary for STOML3 function. (a) Stimulus–response curves for N2a cells overexpressing LifeAct-mCherry and fluorescently tagged STOML3 variants. Data were binned by stimulus magnitude and current amplitudes within each bin averaged for each cell and then averaged between cells, presented as mean±s.e.m; STOML3-V190P-mGFP (magenta squares; 172 measurements, 15 cells), STOML3-R90A-mGFP (grey squares; 218 measurements, 15 cells), STOML3-LR89,90EE-mGFP (green squares; 136 measurements, 13 cells), STOML3-P40S-mGFP (black squares; 142 measurements, 15 cells). Data from wtSTOML3 overexpression are re-plotted here for comparison (cyan squares) (b) Inverted epifluorescent images of STOML3 variants. Note that STOML3-V190P is localized similarly to wtSTOML3; STOML3-R90A and –LR89,90EE are localized in part to the membrane, but the vesicular fraction is lost and STOML3-P40S does not seem to be localized at the membrane nor in a vesicle pool (observations made on 15 cells/4 transfections). Scale bar 10 μm. (c) BiFC assays were used as a cell-based assay for oligomerization. In all cases wtSTOML3-VN was used as bait and as a control wtSTOML3-VC as prey. For experiments conducted on a single day, average slope of YFP signal development for the control was calculated and used to normalize all data. Data are displayed as mean±s.e.m. Oligomerization was significantly reduced when the STOML3-V190P-VC, STOML3-R90A-VC and LR89,90EE-VC variants were used as prey, in comparison with controls; Student’st-test; ***P<0.001;nnumbers indicate the number of transfections. Figure 7: Residues required for oligomerization and correct localization are necessary for STOML3 function. ( a ) Stimulus–response curves for N2a cells overexpressing LifeAct-mCherry and fluorescently tagged STOML3 variants. Data were binned by stimulus magnitude and current amplitudes within each bin averaged for each cell and then averaged between cells, presented as mean±s.e.m; STOML3-V190P-mGFP (magenta squares; 172 measurements, 15 cells), STOML3-R90A-mGFP (grey squares; 218 measurements, 15 cells), STOML3-LR89,90EE-mGFP (green squares; 136 measurements, 13 cells), STOML3-P40S-mGFP (black squares; 142 measurements, 15 cells). Data from wtSTOML3 overexpression are re-plotted here for comparison (cyan squares) ( b ) Inverted epifluorescent images of STOML3 variants. Note that STOML3-V190P is localized similarly to wtSTOML3; STOML3-R90A and –LR89,90EE are localized in part to the membrane, but the vesicular fraction is lost and STOML3-P40S does not seem to be localized at the membrane nor in a vesicle pool (observations made on 15 cells/4 transfections). Scale bar 10 μm. ( c ) BiFC assays were used as a cell-based assay for oligomerization. In all cases wtSTOML3-VN was used as bait and as a control wtSTOML3-VC as prey. For experiments conducted on a single day, average slope of YFP signal development for the control was calculated and used to normalize all data. Data are displayed as mean±s.e.m. Oligomerization was significantly reduced when the STOML3-V190P-VC, STOML3-R90A-VC and LR89,90EE-VC variants were used as prey, in comparison with controls; Student’s t -test; *** P <0.001; n numbers indicate the number of transfections. Full size image We next investigated whether STOML3 sensitization of mechanically gated currents is dependent on the STOML3 stomatin domain. To address this question, we created two protein chimeras: one containing the stomatin domain of stomatin flanked by the amino- and carboxy-terminal regions of STOML3 (Chimera1; Fig. 8 ) and the second containing the stomatin domain from STOML3 flanked by the N- and C-terminal regions of Stomatin (Chimera2; Fig. 8 ). Mechanically gated currents in N2a cells expressing Chimera2 did not differ significantly from those in cells overexpressing wtSTOML3. Chimera1 expression resulted in slightly more sensitive mechanically gated currents compared with those in control N2a cells but this effect was significantly less than that of wtSTOML3 ( Fig. 8 ; Supplementary Fig. 10 ; Supplementary Table 4 ). Thus, the stomatin domain of STOML3 is largely responsible for the effect on Piezo1 sensitivity. 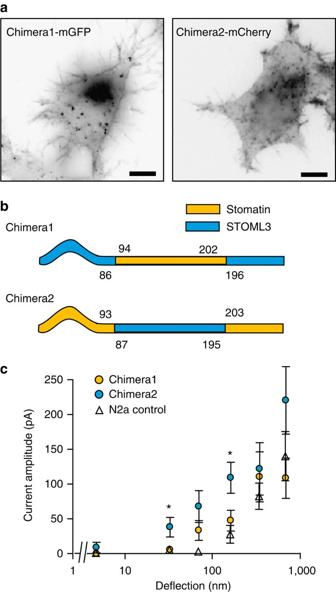Figure 8: The stomatin domain of STOML3 is necessary to sensitize Piezo currents in N2a cells. (a) Inverted epifluorescence images of Chimera1-mGFP and Chimera2-mCherry in N2a cells (observations made in 15 cells/4 transfections and 14 cells/4 transfections respectively; scale bar, 10 μm). Both chimeras localized to a vesicle pool and the plasma membrane. (b) Schematic representation of the two chimera proteins. (c) Stimulus–response data for Chimera1-mGFP (yellow circles; 220 measurements, 15 cells) and Chimera2-mCherry (blue circles; 299 measurements, 14 cells) in N2a cells. Control N2a cell data re-plotted here for comparison (open triangles) Data were binned by stimulus magnitude and current amplitudes within each bin averaged for each cell and then between cells, presented as mean±s.e.m. To test for significance, Student'st-test was used; *P<0.05. Chimera2, containing the stomatin-domain from STOML3, sensitized mechanically mediated currents more effectively than did Chimera1. Figure 8: The stomatin domain of STOML3 is necessary to sensitize Piezo currents in N2a cells. ( a ) Inverted epifluorescence images of Chimera1-mGFP and Chimera2-mCherry in N2a cells (observations made in 15 cells/4 transfections and 14 cells/4 transfections respectively; scale bar, 10 μm). Both chimeras localized to a vesicle pool and the plasma membrane. ( b ) Schematic representation of the two chimera proteins. ( c ) Stimulus–response data for Chimera1-mGFP (yellow circles; 220 measurements, 15 cells) and Chimera2-mCherry (blue circles; 299 measurements, 14 cells) in N2a cells. Control N2a cell data re-plotted here for comparison (open triangles) Data were binned by stimulus magnitude and current amplitudes within each bin averaged for each cell and then between cells, presented as mean±s.e.m. To test for significance, Student's t -test was used; * P <0.05. Chimera2, containing the stomatin-domain from STOML3, sensitized mechanically mediated currents more effectively than did Chimera1. Full size image We have developed a sensitive, quantitative approach to study mechanotransduction in primary sensory neurons that will also be applicable to virtually any adherent cell type. This method was designed such that we could apply fine, measureable physical stimuli at the cell-substrate interface while simultaneously monitoring the electrical response of the cell using a whole-cell patch clamp. We have demonstrated that the most sensitive cellular domain to mechanical stimuli is the cell-substrate interface, as considerably smaller stimuli were required for robust channel gating, in comparison with indentation techniques ( Fig. 2 ). This supports a model in which native mechanotransduction complexes resident in the plasma membrane are linked directly or indirectly to the ECM. This method has enabled us to demonstrate that mechanosensitive ion channels display distinct thresholds depending on the DRG neuronal subtype. Notably, we have identified a class of mechanoreceptors (defined here as type II mechanoreceptors) that display a remarkable sensitivity to mechanical stimuli. Thus, molecular-scale deflections, sometimes less than 10 nm, proved sufficient to gate mechanosensitive channels in these cells. Based on the characteristics of APs measured in type II cells, we suggest that they may be D-hair receptors. We also identified a molecular mechanism controlling the scaling of mechanoreceptor sensitivity: the genetic removal of STOML3 in sensory neurons was sufficient to reduce the sensitivity of almost all mechanoreceptors to a uniformly low level, such that substrate displacements in the order of several hundred nanometres were required to gate mechanosensitive channels in these cells. The dramatic decrease in sensitivity to substrate displacement in the absence of STOML3 probably accounts for the observed mechanoinsensitivity of cutaneous afferents in stoml3 −/− mice [20] . The initiation of AP is dependent on the presence of channels that regulate the excitability of the membrane, like potassium channels [43] , as well as the size of the receptor potentials generated by mechanosensitive channels. We used pillar arrays to study the activation and modulation of Piezo channels, which have been shown to be candidate pore-forming subunits of the mechanosensitive channel in sensory neurons [26] . We show for the first time that a stomatin-domain protein can directly modulate the sensitivity of Piezo1 and Piezo2 channels, shifting the substrate displacement threshold by several orders of magnitude into a range (~10 nm) observed for the native current in ultrasensitive mechanoreceptors. This powerful effect on Piezo channel sensitivity was not found for other stomatin-domain proteins, like stomatin, podocin, MEC-2 and STOML1, and structure–function studies indicated that this activity is primarily located in the stomatin domain of STOML3. The existence of stretch-activated cationic currents in many different cell types has been known for several decades but the molecular identity of these channels has been controversial [18] . The Piezo proteins do form true stretch-activated cation channels and have properties very similar to stretch-activated channel activity recorded in many cell types including sensory neurons [15] , [16] . The question naturally arises as to why cell types with a non-mechanosensory function possess similar stretch-activated channels to specialized mechanoreceptors? There are potentially two answers to this question, which are not mutually exclusive. It may be that the pore-forming subunit of the mechanotransduction apparatus in sensory neurons is not intrinsically stretch sensitive but is rendered so by its association with other proteins, as may be the case for the MEC-4/MEC-10 channels in worm body-touch receptors [24] , [42] . The second possibility is that the mechanosensitivity of stretch-activated pore-forming subunits can be modulated to make them sensitive to mechanical stimuli that are relevant for sensation. We present strong evidence that this latter mechanism indeed operates in mouse sensory neurons. In vivo many mechanoreceptors have remarkable sensitivity, firing APs to skin displacements of less than 1 μm, and this can essentially explain similar psychophysical thresholds to vibratory stimuli [1] , [2] , [43] . We show that the presence of STOML3 in many mouse mechanoreceptors is necessary to ensure that mechanosensitive channels are activated by molecular-scale displacements of the plasma membrane. The magnitude of the mechanical stimulus that reaches mechanoreceptor endings embedded in the skin is likely to be much attenuated compared with stimuli applied to the skin. Thus the nanometre-scale sensitivity is probably necessary to maintain normal psychophysical thresholds for detecting vibration and roughness. The stomatin-domain proteins MEC-2 and STOML3 have both been found to be necessary to maintain mechanoreceptor function in nematodes and mice, respectively [20] , [24] . However, although the MEC-2 protein has been shown to enable the function of constitutively active MEC-4/MEC-10 channels, it has not been shown to induce or modulate an intrinsically mechanosensitive channel [35] , [42] . In contrast, STOML3 can dramatically potentiate the sensitivity of Piezo channels to substrate deflection, but despite modulating a non-DEG/ENaC-type channel, some structural requirements for modulation are similar to those found for MEC-2’s role as part of the mechanotransduction apparatus. Thus mutation of residues involved in cholesterol binding (STOML3-P40S) or those involved in the formation of higher-order oligomerization (STOML3-R90A; STOML3-LR89,90EE) [37] , [38] , [41] , [42] , all abolished the activity of STOML3 and of MEC-2. Some mutant proteins, but not the dimerization mutant V190P, do appear to be mis-localized in cells and therefore it is hard to determine whether oligomerization per se determines correct localization. Interestingly, STOML3 appears to have a highly specific effect as related proteins including, stomatin, STOML1 and MEC-2 did not modulate Piezo1 currents. Nevertheless, STOML3 and STOML1 shared the interesting property of preventing desensitization of channel activity after multiple stimuli at a single pilus. This property may be very important for the in vivo function of such proteins to ensure that mechanoreceptors or nociceptors do not display run-down with repeated stimuli. Indeed, one prominent property of many single afferent fibres in stoml3 −/− -mutant mice is that they respond only once to tap stimulus and cannot subsequently be activated [20] . Using chimeric constructs we show that much of the activity on mechanosensitive currents is apparently retained with the STOML3 stomatin domain. This finding suggests that there is something unique about the STOML3 stomatin domain that enables modulation of mechanosensitive channel gating. We propose that by forming higher-order scaffolds around mechanosensitive channels STOML3 may facilitate the transfer of force to the channel and that mutations that disrupt the ability of STOML3 to form membrane-associated scaffolds disrupt function. Thus, the presence of absolute levels of STOML3 in different receptor types (for example, mechanoreceptors versus nociceptors) may enable the appropriate molecular tuning of mechanoreceptor sensitivity. It is entirely possible that the same mechanism is engaged when nociceptors become sensitized to mechanical stimuli. The method we have introduced offers the opportunity to study molecular-scale gating of mechanosensitive channels with a resolution not previously possible. Cell culture DRGs from C57Bl/6 mice (aged 4–6 weeks, male and female) were dissected and collected in 1 ml phosphate-buffered saline (PBS) on ice and treated with 1 μg ml −1 collagenase IV in 1 ml PBS for 30 min at 37 °C and then treated with 1 ml of 0.05% trypsin in PBS for 5–20 min at 37 °C. Cells were dissociated in 1 ml DMEM/F-12 by passaging with a 20G needle and then collected, washed and finally resuspended in DMEM/F-12 medium containing 10% horse serum and seeded on pillar arrays (2–3 per prep). Cells were cultured overnight at 37 °C in a Steri-Cult 200 incubator with no added neurotrophic factors. Mouse strains from which DRGs were isolated were either wild-type C57Bl/6 from Charles River, or stoml3 −/− on a pure C57Bl/6 background [20] . All experiments involving mice were carried out in accordance with protocols approved by the German federal authorities (State of Berlin). DRG neurons were transfected using the Amaxa Nucleofector Kit, as per the manufacturer’s instructions. Proliferative cells were incubated overnight on pillar arrays, and Fugene HD (Promega) was used for transfection, as per the manufacturer’s instructions. N2a cells (a gift from Phil Selenko) were incubated overnight in media containing low serum (2%) before imaging or patch-clamp analysis. Cultured cell lines (N2a and HEK-293) were tested negative for mycoplasma infection. Molecular biology All fluorescent constructs were generated by replacing EGFP fluorophore of pEGFP-N3 plasmid with a sequence of interest and either monomeric EGFP or mCherry. Constructs for BiFC analysis were created by inserting the gene of interest, in frame, into the multiple cloning site of pBiFC-VC155 or pBiFC-VN173. Point mutations were introduced using PCR-based site-directed mutagenesis. See Supplementary Table 6 for full plasmid list. Fabrication of silicon masters Positive silicon masters were fabricated using standard MEMS technology. Briefly, a silicon wafer of standard thickness (525 μm) was spin coated with a 1-μm-thick layer of positive photoresist (AZ1514). The resist layer was exposed with ultraviolet light and developed. Pillar structures were then created using the BOSCH deep-etching process using a DSE tool from Unaxis. After deep etching, the resist layer was removed. Casting and coating pillar arrays Masters were silanized using vapour phase (tridecafluoro-1,1,2,2-tetrahydrooctyl) trichlorosilane 97% (AB111444, ABCR GmbH & Co. KG, Karlsruhe, Germany) for 8 h. Negative masters were cast from PDMS (Sylgard 184, Dow Corning, USA) using a 1:10 mix of the two components cured at 110 °C for 15 min. The PDMS mould was gently peeled away from the silicon master and the individual arrays were isolated; negative masters were silanized as above and used in four castings before re-silanization [44] . To cast arrays, freshly mixed PDMS (1:10) was placed in a vacuum for 30 min; silanized negative masters were covered with fluid PDMS and left for 30 min. Next, glass coverslips (thickness 2) were activated by oxygen plasma treatment in a FEMTO plasma cleaner (Diener Electronic, Nagold, Germany) and placed, activated side down, on the PDMS-covered moulds. Pillar arrays were cured at 110 °C for 1 h. Two methods were used to coat the pili tops with EHS laminin: reverse microcontact printing and adsorption. PDMS components were mixed at a 1:20 ratio and cured for 15 min at 110 °C and cut into cubits. These cubits were covered with Poly- L -lysine printing ink and incubated for 1 h at 37 °C. The cubits were placed PLL coated side down onto pillar arrays and activated using oxygen plasma treatment. EHS laminin (20 μg ml −1 ) was then adsorbed to the pili for 45 min at room temperature. For adsorption, pillar arrays were silanized and a droplet of EHS laminin (20 μg ml −1 ) was placed in the centre of an array and covered with a glass coverslip to spread the solution. The pillar arrays were then left at 37 °C for 3 h. The second adsorption method gave the most consistent results [45] . All the k =290 pN nm −1 pillar arrays were coated using the adsorption method. Characterizing the mechanical properties of the pillar arrays The elasticity of the same cured PDMS used for pillar arrays was calculated from force-distance curves using an atomic force microscope (Nanowizard II, JPK Instruments AG, Berlin, Germany). SICON cantilevers (silicon, pyramidal-shaped tip, nominal spring constant 0.1–0.6 N m −1 ) were calibrated using JPK software to determine the sensitivity and the spring constant for each experiment. For each sample, at least 250 curves were generated, at 4 distinct points. Force-distance curves were collected in PBS, to eliminate cantilever ‘snap-in’ due to electrostatics. The elasticity of the PDMS was then calculated using the Hertz model, taking into account a pyramidal-shaped indenter with the JPK Instruments analysis software. Scanning electron microscopy (SEM) was used to determine the dimensions of individual elements in the pillar array. Pillar arrays were sputter coated with gold and then imaged either square to or side-on from the array. The diameter of individual pili and the centre–centre distance of the elements were calculated from images taken square to the array. The height of the pili was measured from the images taken perpendicular to the array elements. The spring constant ( k ) of the array elements was calculated from its dimensions and elasticity: where E is the elasticity calculated above. On those occasions when the restoring force required to return the deflected pilus to its central positions was calculated, Hooke’s law was used: where d is the empirically determined deflection of the pilus. Electrophysiology Whole-cell patch-clamp recordings were made using patch pipettes with a tip resistance of 3–7 MΩ, filled with a solution of 110 mM KCl, 10 mM NaCl, 1 mM MgCl 2 , 1 mM EGTA and 10 mM HEPES, adjusted to pH 7.3 with KOH. Extracellular solutions contained (in mM) 140 NaCl, 4 KCl, 2 CaCl 2 , 1 MgCl 2 , 4 glucose and 10 HEPES, adjusted to pH 7.4 with NaOH. We used a Zeiss 200 inverted microscope and an EPC-10 amplifier in combination with Patchmaster software. Data were analysed using Fitmaster software (HEKA Electronik GmbH, Germany). Pipette and membrane capacitance were compensated using the auto function of Patchmaster. Series resistance was compensated by at least 60% to minimize voltage errors. Currents evoked by mechanical stimuli were recorded at a holding potential of −60 mV in sensory neurons, N2a cells and HEK-293 cells. For experiments with sensory neurons, voltage-gated sodium channels were blocked either by a constant superfusion with 1 μM tetrodotoxin or by introducing 10 mM QX-314 in the pipette [6] . Mechanical stimuli were applied by deflecting individual pili using a heat-polished glass pipette (tip diameter 2–5 μm) driven by the MM3A micromanipulator (KleindiekNanotechnik, Germany). In order to generate stimulus–response curves, we applied a series of stimuli over the range of 0–1,000 nm deflection (larger stimuli were excluded). To collect stimulus–response data, the successive stimuli were applied with at least 30-s intervals and the size of each stimulus was randomized. In most cases, more than one pilus per cell was stimulated (see Supplementary Tables 1, 3 and 5 for detailed numbers of cells/stimulation points/stimuli of individual experiments). To collect data on Piezo1 desensitization in N2a cells, increasing stimuli were applied to find a suprathreshold stimulus for that specific cell-matrix region and then successive stimuli of a similar magnitude were applied at 5-s intervals. Bright-field images of pili movement were obtained using a × 40 objective and a CoolSNAP EZ CCD camera (Photometrics, AZ, USA), and the centre of each pilus was determined from a 2D-Gaussian fit of intensity values calculated offline (Igor software, WaveMetrics, USA). To determine movement, successive images were analysed before, during and after deflection. All data points correspond to pillar deflections 0–1,000 nm, with larger deflections discarded. For all data points, the pillar deflection was empirically determined and subsequently plotted against the resulting current amplitude (with an estimated experimental error of 7 nm). In the case of N2a or HEK-293 cells, pili directly underneath the cells were used as stimulation points. In sensory neurons, all sub-neurite stimulation points were within 50 μm of the cell soma (average 23±2.6 μm). We confirmed that distant neurites were under voltage clamp by measuring the reversal potential of SA currents in nociceptors (which was 0 mV at the cell body, n =3) and RA currents in mechanoreceptors (~+60 mV at the as neurite and cell body, n =3). Bimolecular fluorescence complementation For controls, STOML3-VN and STOML3-VC constructs were used as bait and prey. HEK-293 cells were transfected with two plasmids encoding bait and prey proteins using Fugene HD. Transfected cells were then incubated for 8 h in a Steri-Cult 200 incubator. Cells were harvested and resuspended in phenol red-free DMEM media with 25 mM HEPES. For each transfection, a 40 μl cell suspension was dispensed into 24 wells of a 384-well plate. Fluorescence measurements were taken in a plate reader (Infinite 200Pro, TECAN) and relative fluorescence (ex 507±7 nm, em 540±20 nm) was measured every 30 min, at 37 °C. The slope of signal development was used as an indicator of STOML3 oligomerization. BiFC experiments were conducted in triplicate. Real-time qPCR Total RNA was extracted from cells using Trizol treatment and DNA was removed using the Ambion TURBO DNA-free kit. RNA was quantified using a NanoDrop 2000 Spectrophotometer (Thermo Scientific). Two micrograms of RNA per reaction was reverse transcribed with SuperscriptIII Reverse Transciptase (Invitrogen) using random hexamers. With this cDNA, qPCR reactions were performed on a 7900Abi Sequence Detection System (Applied Biosystems) using probes from the Universal Probe Library (Roche). All PCR reactions were conducted in triplicate. Absolute messenger RNA levels were normalized against house-keeping genes HPRT1, cyclophilin D and β-actin. Primers used were as follows: Piezo1, 5′-GACGCCTCACGAGGAAAG-3′ and 5′-GTCGTCATCATCGTCATCGT-3′; Piezo2, 5′-ACGGTCCAGCTTCTCTTCAA-3′ and 5′-CTACTGTTCCGGGTGCTTG-3′; Stoml1, 5′-TCCAGATGGAGAAGCTCAAGA-3′ and 5′-AGCTCTGGTCACGTCATTGAT-3′; and Stoml3, 5′-GGAAGCCAGAGCCAAGGT-3′ and 5′-CATGGAAGCTGACTTCAGAGACT-3′; Hprt1 5′-TCCTCCTCAGACCGCTTTT-3′ and 5′-CCTGGTTCATCATCGCTAATC-3′; cyclophilin D 5′-ATGGTGAAAAACCTGCCAA-3′ and 5′-CATCCTCAGGGAAGTCTGGA-3′; Beta-actin 5′-AAGGCCAACCGTGAAAAGAT-3′ and 5′-gtggtacgaccagaggcatac-3′. Validation of miRNAs Two to three different miRNA sequences per target gene were cloned using the Block-iT Pol II miR RNAi system (Invitrogen). To validate knockdown efficiency, N2a cells were transfected with a plasmid encoding the miRNA and, in the case of STOML3, the STOML3-mCherry plasmid ( Supplementary Table 6 ). After 48 h, total RNA was isolated and reverse transcribed and qPCR experiments were performed. HPRT1 and cyclophilin D were used as the reference genes and a negative control (scrambled miRNA that does not target any known vertebrate gene) was used as a control. The sequence of the selected miRNAs is shown in Supplementary Table 7 . Immunoprecipitation and immunoblotting HEK-293 cells were transiently transfected with two epitope-tagged constructs (STOML3-FLAG with either Piezo1-HA or Piezo2, in a ratio of 1:3) using polyethylenimine (Polyscience). After 24 h, cells were lysed with RIPA buffer (50 mM Tris (pH 7.4), 300 mM NaCl, 1 mM EDTA, 1 mM DTT, 0.5% deoxycholic acid, 0.5% Triton X-100, 0.1% SDS and a protease inhibitor cocktail (Sigma-Aldrich)), incubated for 30 min at 4 °C and centrifuged for 30 min at 13,200 r.p.m. at 4 °C. For immunoprecipitation, 4 μg of monoclonal mouse anti-FLAG antibody (M2 clone, Sigma-Aldrich) was bound to Dynabeads (Dynabeads Protein G, Invitrogen) and samples were processed according to the manufacturer’s instructions. Eluate and lysate of the total protein extract were separated on NuPAGE Novex 3–8% Tris-Acetate Mini-Gels (Invitrogen), blotted on nitrocellulose and subjected to standard antibody detection using the following: mouse monoclonal anti-FLAG antibody (M2 clone, Sigma-Aldrich), mouse monoclonal anti-HA.11 antibody (clone 16B12, Covance), rabbit polyclonal anti-Fam-38b antibody (HPA031974, Sigma-Aldrich), HRP-conjugated goat anti-mouse antibody (ab97265, Abcam) and HRP-conjugated goat anti-rabbit antibody (111-036-003, Jackson ImmunoResearch). Statistical analysis The collection of stimulus–response data generates data sets with variation in both x and y . In order to effectively compare groups for each cell studied, we binned response data by stimulus size in the following bins: 0–10, 10–50, 50–100, 100–250, 250–500 and 500–1,000. For each cell, current amplitudes within each bin were averaged and then bins were averaged between cells. We then tested for significance by testing whether the current amplitude for a given stimulation range (that is, bin) differed between samples. A power analysis was used to determine that moderate to strong effects between samples could be detected with a sample size >4. Most data sets were in excess of this number. All data sets were tested for normality. All normally distributed data sets were compared using a two-tailed Student’s t -test. For nonparametric data, the Mann–Whitney U test was used. In both cases tests were two-sided. In all cases, * P <0.05; ** P <0.01 and *** P <0.001. Categorical data were compared using a χ 2 test. Survival curves were compared using a two-way analysis of variance, and Bonferroni post-tests were used to compare individual points. How to cite this article : Poole, K. et al. Tuning Piezo ion channels to detect molecular-scale movements relevant for fine touch. Nat. Commun. 5:3520 doi: 10.1038/ncomms4520 (2014).